Liquid-metal electrode to enable ultra-low temperature sodium–beta alumina batteries for renewable energy storage Commercial sodium–sulphur or sodium–metal halide batteries typically need an operating temperature of 300–350 °C, and one of the reasons is poor wettability of liquid sodium on the surface of beta alumina. Here we report an alloying strategy that can markedly improve the wetting, which allows the batteries to be operated at much lower temperatures. Our combined experimental and computational studies suggest that addition of caesium to sodium can markedly enhance the wettability. Single cells with Na–Cs alloy anodes exhibit great improvement in cycling life over those with pure sodium anodes at 175 and 150 °C. The cells show good performance even at as low as 95 °C. These results demonstrate that sodium–beta alumina batteries can be operated at much lower temperatures with successfully solving the wetting issue. This work also suggests a strategy to use liquid metals in advanced batteries that can avoid the intrinsic safety issues associated with dendrite formation. Among all types of anode materials, metals such as lithium and sodium have the highest capacity and great potential to increase the energy density of batteries. Unfortunately, these metal anodes have had very limited applications so far in practical devices owing to dendrite formation, passivation of the surface layer and other problems [1] , [2] . Dendrite growth is one of the reasons for safety concerns in current battery devices. One approach to address this problem is to use molten or liquid metal electrodes. This concept has been explored in several types of batteries such as liquid-metal batteries [3] , Li-ion batteries [4] and Na batteries [5] , and successfully used in sodium–beta alumina batteries (NBBs) [6] , [7] , [8] , which are based on a molten sodium anode and β″-Al 2 O 3 solid electrolyte (BASE). Currently, NBBs such as sodium–sulphur (Na–S) battery and sodium–metal halide (ZEBRA) batteries are among the most promising technologies for large-scale renewable energy storage because of their high theoretical specific energy, high energy efficiency and good cycle life [6] , [7] . These technologies have already been in commercial production and widely tested as grid storage and a supplement to wind and solar installations in Japan, France and the United States [9] . However, high operating temperatures (for example, 300–350 °C) are required for battery components to achieve satisfactory electrochemical activity in NBBs. The BASE shows a sufficient ionic conductivity (~0.2 s cm −1 ) for battery applications only at temperatures of 250 °C or above [7] . As for the anode, molten sodium appears to not fully wet the surface of BASE below 400 °C (refs 7 , 10 , 11 ). The poor sodium wetting is one of most challenging issues in NBBs; it is related to formation of a surface oxide film [7] , [10] , [12] , [13] , [14] . Moisture absorbed on the BASE surface could react with sodium to form a surface layer of sodium oxide, which impedes sodium dissolution and sodium ion transport across the sodium anode/BASE interface [12] , [15] , [16] . Impurities such as calcium in the BASE may also deteriorate the sodium wettability during long-term cell cycling [7] , [10] , [14] , [17] . Calcium ions migrate to the interface and form a calcium-oxide film, which blocks contact between the sodium and BASE [18] , [19] , [20] . The high operation temperature significantly increases battery manufacturing and maintenance costs, and causes safety concerns as well. A few safety incidents during the past few years have had a profoundly negative impact on the broad commercialization and implementation of these technologies [21] . Great efforts have been made to modify the sodium anode/BASE interface to improve wetting, such as coating the BASE surface with a thin layer of lead [22] , bismuth [22] or tin [16] , [22] , or adding titanium and aluminium into the sodium anode as oxygen getters [20] , [23] . The combination of these techniques has been proven to successfully eliminate the interfacial effects and resolve the wetting issue at temperatures above 300 °C. However, these techniques appear to be ineffective at lower temperatures, particularly below 200 °C (ref. 24 ). Here we propose a new strategy to enable the use of liquid-metal electrodes at much lower temperatures via alloying. In particular, we develop novel Na alloys, such as Na–K, Na–Rb and Na–Cs as anode materials for NBBs. Computational and experimental studies suggest that these alloys, particularly the Na–Cs alloy, thoroughly change the wetting of sodium on the BASE surface. This strategy is much more effective than any other types of modifications or treatments of the BASE or sodium anode so far, particularly at lower temperatures. Moreover, the addition of these metals to sodium lowers the melting point [25] , [26] , [27] . Therefore, with this technology, new NBBs can be operated at much lower temperatures. Na–S and Na–NiCl 2 cells with the Na–Cs alloy show excellent cycling performance at lower temperatures (for example, 175 and 150 °C). These cells even can be operated at temperature as low as 95 °C with good performance. The reduced operation temperature will simplify battery design/manufacturing and improve battery durability and safety, which eventually will make NBBs competitive with other existing technologies for stationary applications. This work also suggests a new general route of using light-weight liquid metals as electrodes for next-generation safe, high-energy density batteries. Compared with other approaches, such as room-temperature Na- and Li-ion batteries, the NBBs with liquid alloys and dense solid electrolytes will not have issues such as dendrite growth, reaction and inter-diffusion between cell components and so on. Wetting behaviour of Na and Na alloys on BASE surface The new concept is based on the fact that wetting between different surfaces is generally affected by surface energy. The surface energy and wetting are sensitive to atomic composition near the interface. 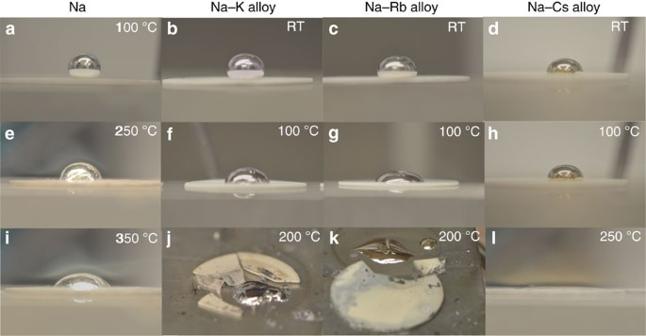Figure 1: Wetting behaviour of Na and Na alloys on BASE surface. (a,e,i) Liquid Na drops on untreated BASE. (b,f,j) Liquid Na–K alloy (molar ratio of 3:7) on untreated BASE. (c,g,k) Liquid Na–Rb alloy (molar ratio of 1:4) on untreated BASE. (d,h,l) Liquid Na–Cs alloy (molar ratio of 1:4) drops on untreated BASE. Figure 1 shows images of pure Na and various types of Na alloys on pristine or untreated BASE at various temperatures. Pure sodium did not wet the untreated surface at 100 °C, but formed a compact liquid droplet, as shown in Fig. 1a . Although the wetting gradually improved with temperature, full wetting on the fresh surface was not observed at temperatures below 400 °C. For example, the contact angle was as high as 52° at 350 °C (see Fig. 1i ; Table 1 ), indicating incomplete wetting of pure sodium on the untreated BASE, which is in agreement with the literature [7] , [10] . Compared with pure sodium, significant improvement in wettability was achieved for Na alloys, as shown in Fig. 1 . Even at room temperature, wetting improved gradually from Na–K, to Na–Rb, to Na–Cs. At 100 °C, all three alloys showed partial wetting on the fresh BASE with contact angles of 91°, 62.4° and 88.6°, which are comparable to that of pure sodium at 250 °C. When heated to 200 °C, the BASE samples coated with Na–K and Na–Rb alloys were fractured (see Fig. 1j,k ). This might be due to ion exchange of Na + by K + and Rb + , considering that K + and Rb + are only slightly larger than Na + (1.33 and 1.47 versus 0.97 Å). Direct replacement of Na + by K + and Rb + has been observed via treatment of beta alumina with the corresponding molten nitrates [28] . The ion exchange in a polycrystalline body typically causes permanent stresses at the grain boundaries due to changes in crystal axis dimensions [28] , [29] , which might be responsible for the observed fracture in the current study. Figure 1: Wetting behaviour of Na and Na alloys on BASE surface. ( a , e , i ) Liquid Na drops on untreated BASE. ( b , f , j ) Liquid Na–K alloy (molar ratio of 3:7) on untreated BASE. ( c , g , k ) Liquid Na–Rb alloy (molar ratio of 1:4) on untreated BASE. ( d , h , l ) Liquid Na–Cs alloy (molar ratio of 1:4) drops on untreated BASE. Full size image Table 1 Contact angles (°) calculated from Fig. 1 and Supplementary Fig. 1 . Full size table As for Cs + , the equilibrium is unfavourable for direct replacement of Na + by Cs + in beta alumina due to the significantly larger size of Cs + (1.69 Å). As a result, no fracture or crack was observed for the BASE sample coated with Na–Cs alloy even heated to 350 °C. The liquid Na–Cs spread over the entire surface at 250 °C with a contact angle of ~0° (see Fig. 1l ), indicating complete wetting on the surface. The detailed wetting behaviour for the Na–Cs alloy is compared with pure sodium ( Supplementary Fig. 1 ) and the corresponding contact angles are listed in Table 1 . It can be seen that the wettability of sodium on the untreated BASE was thoroughly changed with the addition of caesium. When caesium was added to sodium, similar wetting performance was achieved at a temperature at least 150 °C lower, as shown in Table 1 . Once the Na–Cs alloy was wetting the BASE surface at higher temperatures, the wetting behaviour would be maintained even after the sample was cooled down to room temperature, which was similar to that of pure sodium [7] , [10] . As mentioned earlier, coating the BASE surface with a thin layer of lead [22] , bismuth [22] or tin [16] , [22] is typically carried out to improve the wetting. In the current study, the addition of caesium into sodium seemed more effective than these treatments, as compared in Supplementary Fig. 1 . The observed sodium-oxide film ( Supplementary Fig. 1c ) was due to reaction between sodium and Pb/PbO coating on the BASE. As mentioned in the experimental section, the BASE surface was coated with lead acetate aqueous solution and the coating decomposed to lead oxide following heat treatment. The lead oxide reacted with sodium to form a sodium-oxide surface layer during wetting tests. As discussed previously, the incomplete wetting of sodium on the BASE surface is likely related to surface moisture and formation of an oxide film [7] , [10] , [12] , [13] , [14] . Titanium or aluminium is typically added to sodium as an oxygen getter to minimize the formation of sodium oxide at the interface and improve wetting [20] , [23] . This type of explanation may not be applicable to potassium, rubidium and caesium. As shown in Supplementary Table 1 , the standard Gibbs free energies of formation of K 2 O, Rb 2 O and Cs 2 O are −322.1, −294.3 and −327.2 kJ mol −1 , respectively ( http://bachiller.sabuco.com/fq/quimica/tablas-entalpias-inorganicos.pdf ) ( http://kinetics.nist.gov/janaf/ ). They are higher than those for Na 2 O and CaO (compared in Supplementary Table 1 ), which means these oxides are less stable than the latter two. This trend of Gibbs free energies also can be applied at high temperatures ( http://kinetics.nist.gov/janaf/ ). Therefore, potassium, rubidium or caesium cannot act as oxygen getters like titanium or aluminium, and react with Na 2 O or CaO to form the corresponding metal oxides. We conclude that the addition of these metals into sodium is unlikely to break down the oxide film on the BASE. Computational modelling of wetting process To get fundamental insight into the mechanism towards the improved wetting via alloying, simulation of the wetting process was carried out with the Na–Cs alloy. Fifty-atom clusters of sodium or Na–Cs alloy were taken from the initial configuration in their crystal bulk structures. Droplets containing the clusters were set on BASE substrate until equilibrium at various temperatures. Images of the droplets after equilibrium are shown in Fig. 2 ; Supplementary Fig. 2 . 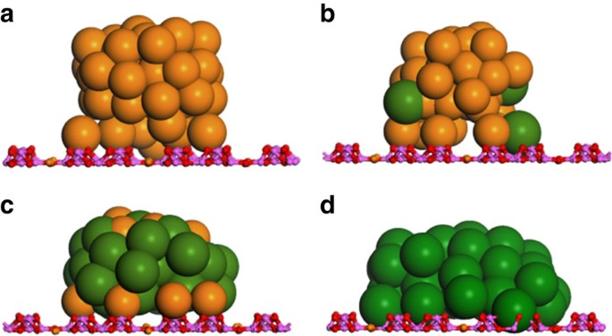Figure 2: Simulated structures of liquid Na–Cs alloy droplets on BASE at 100 °C. (a) Na, (b) Na–Cs (molar ratio of 4:1), (c) Na–Cs (molar ratio of 1:4) and (d) Cs liquid. The Al, O, Na and Cs are coloured purple, red, orange and dark green, respectively. The larger ball of Na and Cs in the droplets is used for graphical purpose. Corresponding heights and widths of the droplets were measured and are listed in Supplementary Table 2 . It can be seen that the height decreased while width increased with higher caesium content in the droplets, which clearly indicated that the wetting gradually improved with the increase of caesium concentration in the alloys. These results were generally in agreement with our experimental observations with various Na–Cs alloy compositions, particularly at 150 °C ( Supplementary Fig. 3 ). Figure 2: Simulated structures of liquid Na–Cs alloy droplets on BASE at 100 °C. ( a ) Na, ( b ) Na–Cs (molar ratio of 4:1), ( c ) Na–Cs (molar ratio of 1:4) and ( d ) Cs liquid. The Al, O, Na and Cs are coloured purple, red, orange and dark green, respectively. The larger ball of Na and Cs in the droplets is used for graphical purpose. Full size image Theoretically, wettability of a liquid-metal droplet on a solid surface can be determined by the work of adhesion, W adh defined as [30] where γ S , γ M and γ I are surface energies of solid-surface vacuum (S), liquid-metal vacuum (M) and interfacial energy of liquid-metal–solid-surface (I). According to the Young–Dupré equation [30] , Therefore, better wettability (that is, smaller contact angle, θ ) is directly related to a larger ratio of W adh / γ M . Compared with sodium ( γ Na =~150 dyn cm −1 ), the surface tension of liquid caesium metal is much lower ( γ Cs =~60 dyn cm −1 ) in the studied temperature range [31] . The calculated W adh for the caesium/β″-alumina system is 121.9 dyn cm −1 , which is larger than that for the sodium/β″-alumina system (65.3 dyn cm −1 ), based on the stronger interactions between caesium and β″-alumina atoms. The larger W adh and smaller γ M for caesium means a smaller wetting angle and, therefore, better wettability on the β″-alumina surface than sodium, as observed in the current study. As evidence, the interface between the BASE and Na–Cs alloy after wetting tests was analysed using scanning electron microscopy/energy-dispersive X-ray spectrometry (SEM/EDS) ( Supplementary Fig. 4 ). The EDS line scan was performed from the BASE/Na–Cs alloy interface (left) to the alloy surface (right). From the EDS line scan, it can be seen that caesium concentration in the anode gradually deceased from the BASE/alloy interface to the alloy surface while the opposite trend was observed for sodium. More detailed chemical composition along the line scan is listed in the Table. All of these results generally agreed with our simulation results that interactions between caesium and β″-alumina atoms are stronger than those between sodium and β″-alumina atoms, and more caesium atoms tend to distribute at the interface. This type of explanation can also be applied to the improved wetting of Na–K and Na–Rb alloys on BASE (refer to Fig. 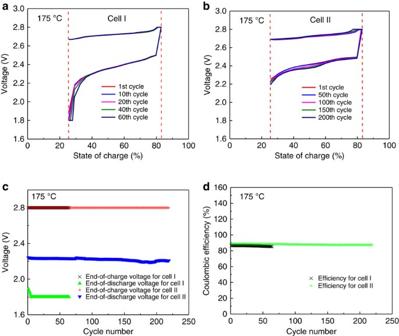Figure 3: Electrochemical cell performance. Cell I: Na|Pb-treated BASE|NiCl2with NaAlCl4. Cell II: Na–Cs|untreated BASE|NiCl2with NaAlCl4. (a) Cell voltage profiles for cell I during the 1st, 10th, 20th, 40th and 60th cycles at 175 °C. (b) Cell voltage profiles for cell II during the 1st, 50th, 100th, 150th and 200th cycles at 175 °C. (c) End-of-charge and -discharge voltage for cells I and II during cycling. (d) Coulombic efficiency for cells I and II during cycling. 1 ), considering their lower surface tension [31] and larger W adh ( Supplementary Table 3 ). Electrochemical cell performance with Na–Cs alloy To further investigate the performance of the Na–Cs alloy as anode material for NBBs, single cells with the Na–Cs alloy anode and untreated BASE were evaluated and compared with those with pure sodium and treated BASE. Figure 3 shows the cycling performance of Na–NiCl 2 cells with Na–Cs and pure sodium anodes at 175 °C. The cells were cycled between 26 and 83% of cell capacity (for example, 160 mAh), as described previously [24] . The SOC (state of charge) of 26–83% was selected based on the fact that, when the cell is overcharged to an SOC of 80% or above, the cell voltage is typically around 2.8 V or higher, and the overcharge may lead to electrochemical reactions between Ni and NaAlCl 4 catholyte, which eventually will cause battery performance degradation during long-term cycling [7] . If the cell is overdischarged to an SOC of lower than 20%, high cell resistance may be incurred at the end of discharge due to insufficient sodium for electrical contact between sodium and the BASE active surface. According to our previous results, the cycling window gradually shifted to the more discharged state due to higher cell resistance at 175 °C (ref. 24 ). Therefore, in the current study, the cells were cycled in a two-step charge/discharge process to maintain the capacity window. The first-step charge was under a constant current of 20 mA (C/4.5), and once the voltage reached 2.8 V, the second step was started under a constant voltage of 2.8 V until a total capacity of 90 mAh was reached. The two-step discharge was similar, including one step under a constant current of 30 mA, followed by a second step at a constant voltage of 1.8 V. Figure 3: Electrochemical cell performance. Cell I: Na|Pb-treated BASE|NiCl 2 with NaAlCl 4 . Cell II: Na–Cs|untreated BASE|NiCl 2 with NaAlCl 4 . ( a ) Cell voltage profiles for cell I during the 1st, 10th, 20th, 40th and 60th cycles at 175 °C. ( b ) Cell voltage profiles for cell II during the 1st, 50th, 100th, 150th and 200th cycles at 175 °C. ( c ) End-of-charge and -discharge voltage for cells I and II during cycling. ( d ) Coulombic efficiency for cells I and II during cycling. Full size image As can be seen in Fig. 3a,b , the charge profiles for both cells were identical, while significant differences were observed at the end of discharge. The end-of-discharge voltage for the cell with the Na–Cs alloy anode was ~2.2 V and remained stable over 200 cycles (see Fig. 3c ), while a precipitous voltage drop at the end of discharge was observed for the cell with the pure sodium anode. The end-of-discharge voltage started at 1.9 V and rapidly decreased to 1.8 V in the first five cycles. Further decrease in the voltage caused the second-step discharge involved. As discussed previously, the precipitous voltage drop was related to either diffusion limitation in the NaAlCl 4 catholyte or poor sodium wetting in the anode at low temperatures [24] . Since the main differences between the current two cells were different anodes along with treated or untreated BASE (that is, sodium wettability), it can be concluded that the gradual voltage drop at the end of discharge in Fig. 3a was due to insufficient wetting on the lead-treated BASE with cycling. For the cell with the Na–Cs alloy anode, however, the end-of-discharge voltage was stable over 200 cycles with negligible degradation. This clearly demonstrated that, in addition to the initial wetting performance, excellent cycle life was achieved in Na–NiCl 2 cells with the Na–Cs alloy as anode material. As discussed earlier in the description of the wetting tests, it was believed that there was no ion exchange between Na + and Cs + due to the significantly larger size of Cs + than Na + (that is, 1.69 versus 0.97 Å). To verify that, we have run post analysis of the cell after 200 cycles and a cross-section of the BASE was analysed using SEM/EDS. As shown in Supplementary Fig. 5 , no Cs was detected in the BASE after long-term operation, which therefore confirmed that there was no exchange between Cs + and Na + . The performance of a Na–Cs alloy anode was also demonstrated for a Na–S battery. Previously, we reported an intermediate-temperature (that is, 150 °C) Na–S battery that uses pure sodium as the anode, BASE as the electrolyte separator and tetraglyme as the catholyte solvent [32] . The cell showed significant improvement in cycle life over state-of-the-art low- or room-temperature Na–S batteries because of the dense ceramic membrane [32] , [33] . 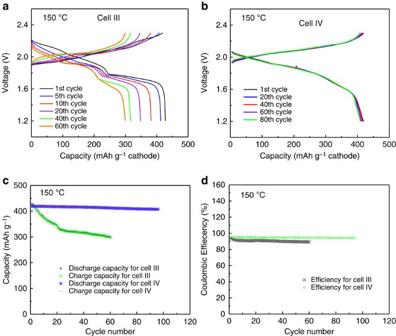Figure 4: Electrochemical cell performance. Cell III: Na|Pb-treated BASE|S with tetraglyme plus 1 M NaI. Cell IV: Na–Cs|untreated BASE|S with tetraglyme plus 1 M NaI. (a) Cell voltage profiles for cell III during the 1st, 5th, 10th, 20th, 40th and 60th cycles at 150 °C. (b) Cell voltage profiles for cell IV during the 1st, 20th, 40th, 60th and 80th cycles at 150 °C. (c) Discharge/charge capacities for cells III and IV during cycling. (d) Coulombic efficiency for cells III and IV during cycling. Figure 4 compares the performance of Na–S cells with Na–Cs alloy and pure sodium anodes. The cells were cycled under constant current of 7 mA (=2.33 mA cm −2 ) with the cutoff voltage between 1.2 and 2.3 V. It can be seen that the initial charge/discharge profiles for both cells at 7 mA (that is,~C/8) were similar, with a capacity of ~420 mAh g −1 ; however, substantial change in cell voltage was observed for the cell with the pure sodium anode and Pb-treated BASE during long-term cycling, which was similar to the observations in the Na–NiCl 2 cell ( Fig. 3a,c ). The charge/discharge cycling in the Na–S cells was controlled by the voltage limit, so the change in voltage caused capacity fade with time. As seen in Fig. 4a,c , >30% of the capacity fade was observed for the Na–S cell with the sodium anode and Pb-treated BASE during 60 cycles. However, the cell with the Na–Cs alloy anode only showed slight degradation, with a capacity fade rate of <3% over 100 cycles ( Fig. 4b,c ). These observations were in agreement with those for the Na–NiCl 2 cell, indicating significant improvement in sodium wettability and cell stability at lower temperatures when pure sodium was replaced with the Na–Cs alloy. Figure 4: Electrochemical cell performance. Cell III: Na|Pb-treated BASE|S with tetraglyme plus 1 M NaI. Cell IV: Na–Cs|untreated BASE|S with tetraglyme plus 1 M NaI. ( a ) Cell voltage profiles for cell III during the 1st, 5th, 10th, 20th, 40th and 60th cycles at 150 °C. ( b ) Cell voltage profiles for cell IV during the 1st, 20th, 40th, 60th and 80th cycles at 150 °C. ( c ) Discharge/charge capacities for cells III and IV during cycling. ( d ) Coulombic efficiency for cells III and IV during cycling. Full size image It is shown that, even with 10 mol% caesium in the alloy, the melting point decreases from 98 to 80 °C (refs 25 , 26 , 27 ). Therefore, by using the novel Na–Cs alloy as the anode, NBBs can potentially be operated at temperatures below 100 °C. Here, we further demonstrated the performance of NBBs with Na–Cs alloy anode at 95 °C. 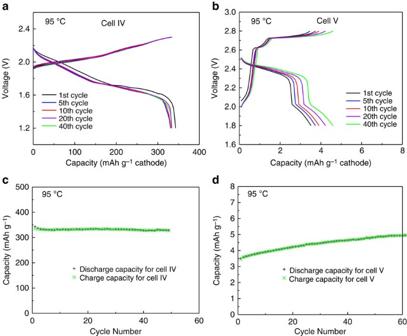Figure 5: Electrochemical cell performance. Cell IV: Na–Cs|untreated BASE|S with tetraglyme plus 1 M NaI. Cell V: Na–Cs|untreated BASE|NiCl2with NaCl-saturated AlCl3-[MEI]Cl. (a) Cell voltage profiles for cell IV during the 1st, 5th, 10th, 20th and 40th cycles at 95 °C. (b) Cell voltage profiles for cell V during the 1st, 5th, 10th, 20th and 40th cycles at 95 °C. (c) Discharge/charge capacities for cell IV during cycling. (d) Discharge/charge capacities for cell V during cycling. Figure 5 shows the performance of Na–S and Na–NiCl 2 cells with the alloy anode. Amazingly, the Na–S cell could be cycled under a constant current of 7 mA (that is, ~C/7) with a high capacity of 330 mAh g −1 (see Fig. 5a ). This high capacity was attributed to the good electrochemical performance of the Na–Cs alloy anode, the BASE and the tetraglyme (with 1 M NaI) catholyte at temperatures below 100 °C. Moreover, the cell showed excellent stability with slight degradation in cell capacity during the initial few cycles and almost no change thereafter, as shown in Fig. 5c . Figure 5: Electrochemical cell performance. Cell IV: Na–Cs|untreated BASE|S with tetraglyme plus 1 M NaI. Cell V: Na–Cs|untreated BASE|NiCl 2 with NaCl-saturated AlCl 3 -[MEI]Cl. ( a ) Cell voltage profiles for cell IV during the 1st, 5th, 10th, 20th and 40th cycles at 95 °C. ( b ) Cell voltage profiles for cell V during the 1st, 5th, 10th, 20th and 40th cycles at 95 °C. ( c ) Discharge/charge capacities for cell IV during cycling. ( d ) Discharge/charge capacities for cell V during cycling. Full size image Owing to the relatively high melting point of NaAlCl 4 (that is, 157 °C), it cannot be used as the catholyte for Na–NiCl 2 battery below 100 °C. Instead, NaCl-saturated AlCl 3 -1-methyl-3-ethylimidazolium chloride (AlCl 3 -[MEI]Cl) [34] , [35] was employed as the catholyte to operate a Na–NiCl 2 cell with a Na–Cs alloy anode at these temperatures. Figure 5b shows the performance of the cell with Na–Cs alloy anode and AlCl 3 -[MEI]Cl catholyte at 95 °C. Unfortunately, the cell showed much inferior performance when compared with the Na–S cell at the same temperature. The initial cell capacity under a constant current of 1 mA was only 3.5 mAh g −1 , and although it gradually increased with cycling, it was still two orders of magnitude lower than that of the Na–S cell (compare Fig. 5a,b ). The low performance in the Na–NiCl 2 cell might be related to insufficient electrochemical activity (for example, ionic conductivity) of the AlCl 3 -[MEI]Cl catholyte compared to tetraglyme with 1 M NaI in the Na–S cell, considering that both cells had an identical anode and electrolyte. Further optimization of the AlCl 3 -[MEI]Cl catholyte is critical to achieve desirable performance of a Na–NiCl 2 battery at these lower temperatures. It should be emphasized that a Na–Cs alloy with a Cs content of 80 mol% was selected for wetting tests ( Fig. 1 ; Supplementary Fig. 1 ), while there was much less Cs in the alloy anodes of single cells. For example, a thin layer of liquid Na–Cs alloy (80 mol% Cs) was initially coated on the BASE for Na–NiCl 2 cells during fabrication. During first charge, Ni reacted with NaCl in the cathode and sodium was gradually generated at the anode side. After full charging, the alloy in the anode had only 6.7 mol% Cs ( Supplementary Fig. 6 ). When the cells were cycled at an SOC of 26–83%, the Cs content in the alloy was between 20.8 and 7.9 mol%. For Na–S cells, since they were started in a fully charged state, an alloy with 6.7 mol% Cs was loaded into the anode chamber during assembly and the cells were cycled in a similar SOC window with a similar amount of Cs in the anode. In additional to the cell performance, we have further tested wettability of an alloy with 5 mol% Cs (Na:Cs ratio of 95:5). As seen in Supplementary Fig. 3 , the wetting was still much better than pure sodium at 100 °C, which was consistent with the cell-testing results. On the basis of these discussions, it can be concluded that Cs content in the alloy anode was not necessarily maintained at 80 mol%, as it was in the wetting measurements. Considering the high cost of caesium metal, with less caesium addition to the anode, the overall material cost of these novel NBBs will be reduced and comparable with the state-of-the-art NBBs. In conclusion, addition of caesium to sodium markedly improves its wettability on the surface of BASE. According to our computational and experimental studies, the improvement is related to lower surface tension of liquid caesium metal, and stronger interactions between Cs and β″-alumina atoms compared with those with sodium. Single cells with Na–Cs alloy anodes also show marked improvement in cycle life over those with pure sodium anodes. This study implies that the wetting issue in NBBs can be markedly suppressed via addition of other metals such as caesium to the sodium anode. Of course, successful operation of NBBs with high performance at lower temperatures requires us to further address other problems, such as BASE resistance and polarization in the cathodes. This work may also suggest a new approach of using liquid-metal anode and impermeable solid electrolyte for next-generation high-performance batteries, which are intrinsically safer than state-of-the-art room-temperature batteries. BASE fabrication BASE discs were prepared using a vapour phase process as described previously [7] , [24] , [32] , [36] , [37] . α-Al 2 O 3 (Almatis, >99.8%), yttria-stabilized zirconia (YSZ) (8YSZ, UCM Advanced Ceramics), dispersant (Phospholan PS-236, Akzo Nobel), solvent (methyl ethyl ketone/ethanol), plasticizer (benzyl butyl phthalate, Aldrich), and binder (Butvar B-79) were thoroughly mixed to make a slurry. The slurry was cast into thin sheets, and the sheets were laminated and laser-cut into circular discs. The discs were fired at 1,600 °C in air to achieve full density (>99%). The sintered α-Al 2 O 3 /YSZ discs then were placed in a loose β″-Al 2 O 3 powder and heat-treated at 1,450 °C in air to convert α-Al 2 O 3 into β″-Al 2 O 3 . The β″-Al 2 O 3 powder used for the conversion process was synthesized separately via a solid-state reaction [7] . The thickness of the converted composite β″-Al 2 O 3 /YSZ discs was ~600 μm. Wettability test The sessile drop technique was used to measure the contact angle of liquid sodium or sodium alloys on the BASE surface, as described previously [16] . High-purity Na (Alfa Aesar, 99.95%), K (Alfa Aesar, 99.96%), Rb (Alfa Aesar, 99.95%) and Cs (Alfa Aesar, 99.98%) were selected as the starting materials. The as-received BASE samples without any surface modifications or treatments were heated on a hot plate in an argon-protected glove box to the desired temperatures. Some BASE samples coated with lead were also tested for comparison. During the process, the BASE surface was first coated with saturated lead acetate aqueous solution and then heat-treated in an argon-protected atmosphere at 400 °C to decompose the lead acetate to lead oxide, which was reduced to lead metal during testing. Pure sodium or sodium alloys were heated to the testing temperatures and drops of the liquid metal were transferred to the surface of the BASE using a glass pipette. The wettability test was carried out in a temperature range from room temperature to up to 350 °C with a holding time of 30 min at each temperature for wetting-angle measurements. Computational modelling Ab initio molecular dynamics simulations were carried out using the density functional theory with a spin-polarized gradient-corrected functional for exchange and correlation as implemented in the CP2K software package ( www.cp2k.org .) [38] , [39] , [40] . The wave functions were expanded in a double-zeta Gaussian basis set [41] . An auxiliary plane-wave basis [42] with 480 Ry energy cutoff was used in the calculation of the electrostatic energy terms. Core electrons were modelled by scalar relativistic norm-conserving pseudopotentials [43] , [44] , [45] and the Г-point approximation was employed for Brillouin zone integration. All ab initio molecular dynamics simulations were performed by sampling the canonical (NVT) ensemble employing Nose–Hoover thermostats [46] , [47] . After the equilibration phase of 3.0~5.0 ps (depending on the temperature), the well-equilibrated structure at the specific temperature was analysed. The liquid-metal or alloy droplet over β″-alumina substrate was modelled with a fifty-atom metal or alloy cluster (Na 50 , Cs 50 , Na 40 Cs 10 and Na 10 Cs 40 ) interacting with the periodic β″-alumina surface slab. All periodic simulation systems included a 30-Å vacuum layer between periodic images in the Z direction. The initial configurations of the metal or alloy clusters were taken from their crystal bulk structures. The β″-alumina used in the simulation had a slab size of 29.2593 × 33.4500 × 5.6300 Å and a composition of Na 30 Al 198 O 306 . A qualitative description of the wettability can be given by height of the droplet (pseudo-spherical) and width (diameter) of the interfacial area (pseudo-circular). Considering the large size difference between Na and Cs atoms (Cs:Na=1.43) [25] , [26] , [27] , the comparable heights and widths of Na and Na-rich droplets were scaled by a factor of 1.43. Catholyte synthesis In the current study, a catholyte of NaAlCl 4 was used when the Na–NiCl 2 battery was operated at 175 °C. NaAlCl 4 was synthesized by mixing NaCl (Alfa Aesar, 99.95%) and AlCl 3 (Alfa Aesar, 99.99%) with a molar ratio of 1.15:1, followed by heat treatment at 320 °C in an argon-filled glove box. A room-temperature molten salt of NaCl-saturated AlCl 3 -1-methyl-3-ethylimidazolium chloride ([MEI]Cl) was selected as the catholyte for Na–NiCl 2 batteries operated at 150 °C or lower [34] , [35] . It was prepared by mixing AlCl 3 (Alfa Aesar, 99.99%) and [MEI]Cl (Alfa Aesar, 99.99%) with a molar ratio of 4:1 at 150 °C in the argon-filled glove box. The melt was purified by immersing Al foil (Alfa Aesar, 99.99%) into the melt. Excess anhydrous NaCl (Alfa Aesar, 99.99%) was then added into the melt and heated at the same temperature overnight. For the Na–S battery, tetraglyme containing 1 mol NaI was selected as the catholyte as before [32] . Cell construction and testing Single cells were fabricated as described previously [24] , [32] , [36] , [37] . BASE discs with a diameter of 26 mm were glass-sealed to α-Al 2 O 3 rings with an active cell area of ~3 cm 2 . Some of the glass-sealed α-Al 2 O 3 rings were further treated by coating the anode side of the BASE surface with a thin layer of lead. The cell assembly then was moved into the argon-filled glove box. For the Na–NiCl 2 battery, 1 g of cathode granules consisting of Ni, NaCl and small amounts of additives were put into the cathode chamber [24] . Molten catholyte of NaAlCl 4 or NaCl-saturated AlCl 3 -[MEI]Cl was infiltrated into the cathode. For the Na–S battery, the catholyte of NaI-containing tetraglyme was heated to 150 °C and a mixture of S and Na 2 S 4 (molar ratio of 4:1) was dissolved into the solution [32] . The solution was poured into the cathode chamber and a carbon felt was inserted into the chamber as a current collector. A foil and spring made of Mo were placed on top of the cathode as a current collector. When liquid Na–Cs alloy was used as the anode, a thin layer of the alloy (0.06 g, molar ratio of 1:4) was brushed onto the surface of pristine BASE. If pure sodium was selected as the anode, a small piece of sodium was preloaded onto the lead-coated BASE for initial contact. For the Na–S battery, since it was assembled in a fully charged state, the desired amount of sodium or Na–Cs alloy was added into the anode chamber during assembly. A spring-loaded stainless steel shim was inserted into the compartment as molten sodium reservoir. Anode and cathode end plates were then compression-sealed to both sides of the α-Al 2 O 3 ring using silver O-rings. Nickel leads, which served as current collectors, were welded to the electrode end plates. The assembled cells were heated in air to the desired temperatures. The galvanostatic discharge/charge test was carried out with a BT-2000 Arbin Battery Testing system as before [24] , [32] , [36] , [37] . How to cite this article: Lu, X. et al . Liquid-metal electrode to enable ultra-low temperature sodium–beta alumina batteries for renewable energy storage. Nat. Commun. 5:4578 doi: 10.1038/ncomms5578 (2014).